Vertical twinning of the Dirac cone at the interface between topological insulators and semiconductors Topological insulators are a new class of matter characterized by the unique electronic properties of an insulating bulk and metallic boundaries arising from non-trivial bulk band topology. While the surfaces of topological insulators have been well studied, the interface between topological insulators and semiconductors may not only be more technologically relevant, but the interaction with non-topological states may fundamentally alter the physics. Here, we present a general model to show that this type of interaction can lead to vertical twinning of the Dirac cone, whereby the hybridized non-spin-degenerate interfacial states cross twice as they span the bulk bandgap. This hybridization leads to spin–momentum locking of non-topological states with either helical (clockwise or anticlockwise) or even anti-helical (negative winding number) spin orientation depending on the parametization of the interaction. Model results are corroborated by first-principles calculations of the technologically relevant Bi 2 Se 3 film van der Waals bound to a Se-treated GaAs substrate. Topological insulators (TIs) are somewhat unique in the history of condensed matter physics, as both the nature of these materials and many of their associated exotic properties were predicted on purely theoretical grounds before experimental evidence of their existence was found [1] , [2] , [3] . The topology of an insulator is associated with the continuous deformation of its Hamiltonian; if it can be continuously deformed to yield the band structure of another insulating system, while maintaining a bandgap throughout the deformation, then they belong to the same topological group and have the same associated Z 2 topological invariant [2] . The relatively small bandgap and large spin–orbit interaction in TIs lead to the non-trivial topology and a Z 2 invariant, which is distinct from normal insulators (NIs) such as GaAs, Si or even vacuum. Although the bulk properties of TIs are similar to ordinary insulators, the interface between two materials with different topological invariants leads to the emergence of a topologically protected metallic state, which is localized to the interface and has a linear Dirac-cone-like dispersion relation, as described in the Kane–Mele model [1] , [4] , [5] . Although most current studies are focused on TI surfaces [6] , [7] , [8] , [9] , [10] , [11] , this represents only a special case of all possible interfaces, that is, the interface with vacuum. Despite being less studied, real interfacial states are not only unavoidable at the substrate, but may be even more advantageous for applications than utilization of the surface states. Interfacial states are protected from the environment, indispensable for creating edge-state electrical circuits, and the formation of periodic heterostructures of TIs and NIs may provide numerous channels for topological current, potentially obtaining bulk-like current densities while maintaining topological protection. Similar to the surface, it is believed that interfacial topological states are spin–momentum locked, where the spin polarization of the electron is locked in plane and perpendicular to the crystal momentum, k , leading to a number of potential applications [11] , [12] . They may find great use in spintronics, as the spin current can now be controlled without magnetism, but instead through the application of electric fields leading to new architectures for spin-based transistors [13] , [14] , [15] . Furthermore, the weak antilocalization of the Dirac state is robust against disorder, and localized non-magnetic perturbations cannot lead to backscattering of the electron, yielding dissipationless transport. The current lack of attention on interface states is not due to their lack of importance, but instead on the experimental difficulty in their characterization. As they are beyond the scope of standard surface-sensitive techniques, little is experimentally known and they have only recently been detected [16] . While the interfacial Dirac cone is generally believed to have essentially identical characteristics to that of the surface, we note that due to the large difference in ionization energies among promising TIs (such as the pnictogen chalcogenides) and ordinary semiconductors, other localized states at the interface may greatly alter the interface properties. Interface states have been studied in a number of contexts: TI/graphene [17] , HgTe/CdTe heterostructure [18] , TI/2D semiconductor [19] and for semiconducting thin films on TI [20] . One of the particularly intruiging predictions on the semiconducting/TI interface state is the possibility that non-topological states can acquire spin texture due to their interaction with the topological interface state [20] . Herein, we construct a simple model Hamiltonian to describe the interaction of the topological interface state with non-topological states and use first-principles density functional theory (DFT) to calculate the band structure and spin texture of the prototypical semiconducting/TI interface, GaAs/Bi 2 Se 3 . We demonstrate that not only can non-topological interface states indeed acquire spin texture, but that in general there exists a change in the helicity of the spin locking of the interfacial states at some critical | k |. In addition, we find that the type of interaction depends strongly on both the band offset between the TI and semiconductor as well as the chemical nature of the interface, suggesting that novel optical and electronic phenomena can be achieved through chemical modification of the interface. Model hamiltonian The pristine TI states at the interface are described by a massless Dirac cone with helical (spin–momentum locked) spin textures represented by the effective surface Hamiltonian, , where v F is the Fermi velocity, k is the wavevector, σ is the Pauli vector and is the unit vector normal to the interface depicted in Fig. 1a . Given that in general TIs have a narrow bulk bandgap, the simplest model would be to consider that the Dirac cone interacts with only a single band of the semiconductor that enters the TI bulk gap as shown in Fig. 1b,c , where Δ is the energy of the conduction band minimum (CBM) or valence band maximum (VBM) relative to the Dirac point. This semiconductor-derived state can be described by a spin-degenerated parabola, , where m * is the effective mass of either the electrons or holes. 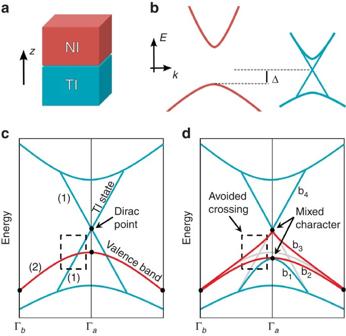Figure 1: TI/NI interface-effective Hamiltonian model. (a) Schematic representation of the interface between a topological insulator (TI) and a normal insulator (NI),zis normal to the interface. (b) The band structures of the semiconductor (shown in red) and topological insulator (shown in blue) are depicted for the case of type-II alignment, whereby the VBM of the semiconductor lies within the bulk gap of the topological insulator. The Δ parameter in the Hamiltonian model is the VBM energy relative to the Dirac point. (c) Band structure at the interface in the absence of mutual interaction between the TI and NI. The topological interface state is shown in blue with linear dispersion and the semiconductor-derived bands are shown in red with parabolic dispersion. The degeneracy of the bands are labelled, either (1) non-degenerate or (2) doubly degenerate, and the black dots indicate points that are required to be doubly degenerate due to the preservation of TRS. The dashed box indicates the region in which the NI state and the TI state cross. (d) The effect tocwhen interaction is turned on. The effect of the interaction is highlighted in the dashed box, in which the interaction leads to an anticrossing between the previously doubly degenerate NI state and the singly degenerate TI state, which requires the interconversion of the character of semiconducting bands and TI bands. As a result, neither of the double degeneracies at Γacan cleanly be labelled as the Dirac point, as both consist of the crossings of state that change from TI to semiconductor character. Using the basis , where are the TIs spinors and are the semiconductor spinors, we can write the interaction between the topological and semiconductor states in k -space as follows, Figure 1: TI/NI interface-effective Hamiltonian model. ( a ) Schematic representation of the interface between a topological insulator (TI) and a normal insulator (NI), z is normal to the interface. ( b ) The band structures of the semiconductor (shown in red) and topological insulator (shown in blue) are depicted for the case of type-II alignment, whereby the VBM of the semiconductor lies within the bulk gap of the topological insulator. The Δ parameter in the Hamiltonian model is the VBM energy relative to the Dirac point. ( c ) Band structure at the interface in the absence of mutual interaction between the TI and NI. The topological interface state is shown in blue with linear dispersion and the semiconductor-derived bands are shown in red with parabolic dispersion. The degeneracy of the bands are labelled, either (1) non-degenerate or (2) doubly degenerate, and the black dots indicate points that are required to be doubly degenerate due to the preservation of TRS. The dashed box indicates the region in which the NI state and the TI state cross. ( d ) The effect to c when interaction is turned on. The effect of the interaction is highlighted in the dashed box, in which the interaction leads to an anticrossing between the previously doubly degenerate NI state and the singly degenerate TI state, which requires the interconversion of the character of semiconducting bands and TI bands. As a result, neither of the double degeneracies at Γ a can cleanly be labelled as the Dirac point, as both consist of the crossings of state that change from TI to semiconductor character. Full size image For the most general type of interaction, the 2 × 2 interaction matrix V int can be expanded in terms of Pauli matrices, where each α is an independent complex parameter. In the absence of interaction, the solutions to equation (1) at the Γ-point leads to two sets of doubly degenerate solutions: those associated with the Dirac point of the topological interface state at E =0 and those of the doubly degenerate semiconductor state at E =Δ. This degeneracy at the Γ-point is the spin degeneracy that is guaranteed by Kramers theorem, whereby operating on the eigenfunction with the time reversal operator (where K represents complex conjugation) yields the eigenfunction of the energy degenerate Kramers pair. It is the time reversal symmetry (TRS) that is said to protect the topological state, as only perturbations that break TRS (such as the presence of magnetic impurities) can break the degeneracy. Herein, however, we focus our attention on perturbations that preserve the TRS, as these are most relevant at the ‘standard’ TI/NI interface in the absence of localized magnetic moments or long-range ordering. This is accomplished by requiring that V int commutes with the time reversal operator, at the time reversely invariant momenta points in the Brillouin zone. This leads to the following constraints for the α -parameters: whereby α 0 must be wholly real and α 1 , α 2 and α 3 are purely imaginary. Solving for the energy eigenvalues of equation (1), we find that indeed interactions of this form preserve the double degeneracy at the Γ-point, with eigenvalues at where we have defined the total magnitude of the interaction, . Upon first glance, not much seems to have changed, with the interaction increasing the energy between the Dirac point and the band edge from Δ to . However, the interaction also leads to an avoided crossing off Γ, as shown schematically in Fig. 1d . While this interaction cannot in principle open a gap, as it is an avoided crossing between the doubly degenerate semiconductor band and the non-degenerate TI state, it necessarily leads to a region where the interaction causes the interconversion of the character of the semiconductor bands and the TI state. Note that the lower branches of the Dirac cone cannot directly join with the upper branch near the Dirac point as they cannot cross the semiconductor band and hence, the lower branch of the TI state becomes degenerate with the bulk-derived state at Γ a . As the degenerate states at Γ become close in energy, neither of these degenerate states can be clearly distinguished as the Dirac point, as both exhibit the evolution of topological states into bulk semiconductor-derived states. To investigate the nature of these mixed states, particularly how the helical nature of the topological interface state is altered under the interaction, we investigate the spin textures of the four bands of the model. In the current basis, the spin textures of the Bloch eigenstates of the effective Hamiltonian are calculated by the expectation values of the 4 × 4 matrices: While as suggested by equation (4), the calculated band structure depends only on the total magnitude of the interaction, α M , the nature of the resulting spin texture is found to be dependent on the details of the interaction and the relative magnitudes of the contributing α i ’s. Spin textures for the four bands for different choices for the non-vanishing interaction parameter α i are shown in Fig. 2 . 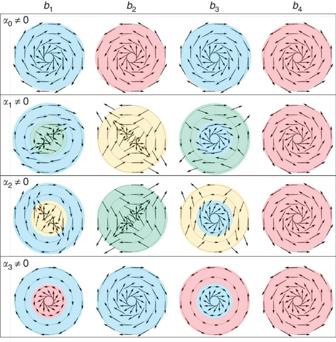Figure 2: Helicity of the bands of the model Hamiltonian. Each figure shows the spin orientation for a particular band for various concentric circles in thekx–kyplane, with the centre being the Γ-point. They are arranged in columns of differing band number, labelled (b1–4) in increasing energy. Each row corresponds to considering a different type of interaction forVint. In each case, we assume thatVintis parameterized by a single parameter and that all of the other parameters vanish. The choice for non-vanishing parameter,αi≠0, is indicated for each row. The blue- and red-shaded regions indicate left- and right-handed spin texture, respectively. The yellow and green regions indicated left- and right-handed anti-helical spin texture, where the spin has a negative winding number. Figure 2: Helicity of the bands of the model Hamiltonian. Each figure shows the spin orientation for a particular band for various concentric circles in the k x – k y plane, with the centre being the Γ-point. They are arranged in columns of differing band number, labelled (b 1–4 ) in increasing energy. Each row corresponds to considering a different type of interaction for V int . In each case, we assume that V int is parameterized by a single parameter and that all of the other parameters vanish. The choice for non-vanishing parameter, α i ≠0, is indicated for each row. The blue- and red-shaded regions indicate left- and right-handed spin texture, respectively. The yellow and green regions indicated left- and right-handed anti-helical spin texture, where the spin has a negative winding number. Full size image There are several interesting features for these spin textures. First, for all cases, all four bands in the model become spin-textured as a result of the interaction. In addition to the helical spin states associated with the TI interface state, interactions containing σ x or σ y terms can induce an anti-helical spin texturing in the bulk-derived band. For these anti-helical states, see for instance the yellow-shaded b 2 under α 1 , as you transverse the Brillouin zone in a anticlockwise direction the spin rotates in a clockwise manner, leading to a winding number of −1. Also interesting is the qualitative change in spin texture for individual bands, for instance b 1 under α 3 , that changes from right-handed (anticlockwise) helical to left-handed (clockwise) helical at some critical | k |. Although strange at first sight, this has a straightforward explanation—it corresponds to a change of character of the bands in the vicinity of an avoided crossing. Note that, if the bulk-derived state has a large curvature, it is possible for it to intersect with the Dirac cone twice instead of only once, leading to three distinct regions of spin texture. Although this second critical | k | is not guaranteed to exist, we mention it here for the sake of completeness. Focusing on those features that are similar irrespective of the type of interaction, we see that the highest energy band, b 4 , keeps its right-handed helical nature under all interactions. This is expected as the semiconductor band intersects with the Dirac cone below the Dirac point, hence the spin texture of the top half of the Dirac cone (b 4 ) remains unchanged. Similarly, near the Dirac point at Γ, b 3 posses the left-handed helicity of the bottom half of the Dirac cone. As we move away from Γ, however, b 3 changes character to that of a semiconducting state, as shown in Fig. 1 . As a result, at large k its helicity can be either left- or right helical or anti-helical, depending on the nature of the interaction between the TI and non-TI states. At larger k , b 1 can be identified as the bottom half of the original Dirac cone, having the same left-handed helicity under all interactions. While the original Dirac point can be seen at Γ, where b 3 and b 4 are degenerate, the second degeneracy (b 1 and b 2 at Γ) also now involves the crossing of non-spin-degenerate interfacial states that do not become degenerate at other time reversely invariant momenta points. As such, this can be viewed as the emergence of a secondary Dirac point within the gap. Furthermore, for interactions parameterized by α 0 or α 3 , the spin texture of b 1 and b 2 will form that of a Dirac cone in the vicinity of Γ. While this can be viewed as the emergence of a secondary Dirac point, it is important to note that it is vertically connected to the original Dirac point through the degeneracy at Γ b , see Fig. 1d . Hence it is the result of hybridization which does not affect the topological classification and its appearance is not associated with a topological phase transition. To find a system that may exhibit the exotic physical properties of the model and shed light on the nature of the interaction, we turn to the technologically relevant Bi 2 Se 3 /GaAs interface. First-principles calculations To construct a realistic atomistic model of the Bi 2 Se 3 /GaAs interface, we use first-principles DFT calculations (see Methods) to first investigate the chemical stability and electronic properties of the isolated Se-treated As-terminated GaAs(111) surface. In the 2 × 2-unit cell, we considered Se replacing between 0 and 4 surface As, yielding 0–1.00 monolayer (ML) of Se coverage: 0, 0.25, 0.50, 0.75 and 1.00 ML. Ball-and-stick models of geometries of GaAs(111) surfaces with a Se treatment of 0.75 ML is shown in Fig. 3a . The chemical stability map for the different Se coverages as a function of the chemical potentials μ Se and μ As is shown in Fig. 3b . We focus our attention first on the 0.75-ML coverage case, as this is the most energetically stable surface for a large range of chemical potentials and leads to a fully passivated GaAs(111) surface, which maintains its bulk bandgap. 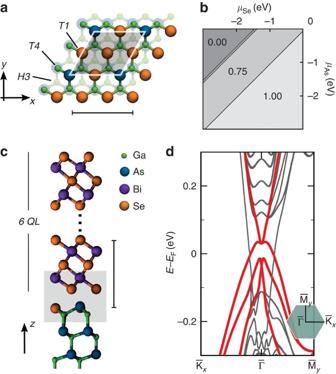Figure 3: First-principles calculations of the Bi2Se3/GaAs interface. (a) Top view of a ball-and-stick model for GaAs(111) surface with 0.75 ML of Se treatment. The unit cell is shaded in grey; scale bar, 5 Å. The stacking sites of the first atomic layer of Bi2Se3are labelled by H3, T4 and T1. (b) Chemical stability map for the GaAs(111) surface. The shaded regions indicate which Se surface coverage of the GaAs(111) surface is the most stable as a function of the chemical potentials of As and Se,μAsandμSe. (c) Side view of a ball-and-stick model for Bi2Se3/GaAs interface with 0.75 ML of Se treatment and H3 stacking. The shaded area shows the interface region; scale bar, 1 nm. (d) Electronic band structure for Bi2Se3/GaAs with 0.75 ML of Se treatment. Four bands near the Fermi level are highlighted in red for comparison with the effective Hamiltonian. Figure 3: First-principles calculations of the Bi 2 Se 3 /GaAs interface. ( a ) Top view of a ball-and-stick model for GaAs(111) surface with 0.75 ML of Se treatment. The unit cell is shaded in grey; scale bar, 5 Å. The stacking sites of the first atomic layer of Bi 2 Se 3 are labelled by H3, T4 and T1. ( b ) Chemical stability map for the GaAs(111) surface. The shaded regions indicate which Se surface coverage of the GaAs(111) surface is the most stable as a function of the chemical potentials of As and Se, μ As and μ Se . ( c ) Side view of a ball-and-stick model for Bi 2 Se 3 /GaAs interface with 0.75 ML of Se treatment and H3 stacking. The shaded area shows the interface region; scale bar, 1 nm. ( d ) Electronic band structure for Bi 2 Se 3 /GaAs with 0.75 ML of Se treatment. Four bands near the Fermi level are highlighted in red for comparison with the effective Hamiltonian. Full size image The interface is constructed by stacking six quintuple layers of Bi 2 Se 3 on the fully passivated 0.75-ML Se-substituted GaAs (111) surface, as shown in Fig. 3c , with the Se from the Se atomic layer of Bi 2 Se 3 directly above the hollow site (H3), which has three nearest neighbours on the substrate, as indicated in Fig. 3a . This was chosen as the Se directly above the tetrahedral site T1 (having a single nearest neighbour on the substrate) or T4 (having four nearest neighbours on the substrate) were found to be 490 and 20 meV per supercell higher in energy, respectively. The calculated band structure of the Bi 2 Se 3 /GaAs interface is shown in Fig. 3d . To identify which states are localized at the interface and originate from the non-trivial band topology, we perform a local real-space projection of each of the eigenfunctions onto the interfacial region shaded in Fig. 3c . The four bands that are most strongly localized to the interfacial region are shown highlighted in red in the band structure. An enlargement of the band structure near the -point and the accompanying spin textures of these four bands, labelled b 1 –b 4 , are shown in Fig. 4a,c , respectively. These four bands are directly comparable to the bands of the model, with b 2 and b 3 originating from the VBM of GaAs and becoming degenerate away from . Furthermore, the spin texture indicates appreciable spin locking in the b 1 , b 2 and b 4 bands. 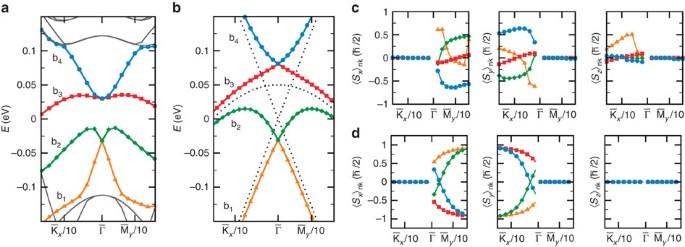Figure 4: First-principles calculations and Hamiltonian model for the 0.75-ML Se-treated Bi2Se3/GaAs interface. (a) An enlarged version near the Γ-point of the first-principles band structure of the Bi2Se3/GaAs interface with 0.75-ML Se coverage. The coloured bands that are labelled b1–b4are the hybridized VBM-derived state and the Dirac cone at the interface, which are directly comparable to the model calculation; other bands shown in grey are addition bands present in the first-principles calculation, which are not considered in the model. (b) Effective model band structure using the interaction parameters (α3=i0.05 eV,α0=α1=α2=0) and calculated material parametersvF=5 × 105ms−1,m*=−0.456m0and Δ=0.05 eV. The dashed lines indicate the band structure from the model in the absence of interaction between the Dirac cone and VBM-derived state. The projections of the spin textures in the vicinity of the-point for the bands b1(orange), b2(green), b3(red) and b4(blue) along the Cartesian directions are shown incanddfor the first-principles calculation and the effective Hamiltonian model, respectively. The reversal of the sign of the projection of a band nearindicates the reversal of the helicity of the spin texture of that band. Figure 4: First-principles calculations and Hamiltonian model for the 0.75-ML Se-treated Bi 2 Se 3 /GaAs interface. ( a ) An enlarged version near the Γ-point of the first-principles band structure of the Bi 2 Se 3 /GaAs interface with 0.75-ML Se coverage. The coloured bands that are labelled b 1 –b 4 are the hybridized VBM-derived state and the Dirac cone at the interface, which are directly comparable to the model calculation; other bands shown in grey are addition bands present in the first-principles calculation, which are not considered in the model. ( b ) Effective model band structure using the interaction parameters ( α 3 = i 0.05 eV, α 0 = α 1 = α 2 =0) and calculated material parameters v F =5 × 10 5 ms −1 , m *=−0.456 m 0 and Δ=0.05 eV. The dashed lines indicate the band structure from the model in the absence of interaction between the Dirac cone and VBM-derived state. The projections of the spin textures in the vicinity of the -point for the bands b 1 (orange), b 2 (green), b 3 (red) and b 4 (blue) along the Cartesian directions are shown in c and d for the first-principles calculation and the effective Hamiltonian model, respectively. The reversal of the sign of the projection of a band near indicates the reversal of the helicity of the spin texture of that band. Full size image To determine how representative the model presented in equation (1) is of the physics at the interface, we independently determine the material parameters for the model from first-principles calculation. We find a Fermi velocity of v F =5 × 10 5 m s −1 for the Dirac cone of the pristine Bi 2 Se 3 , an effective mass of m *=−0.456 m 0 for the heavy holes of the GaAs surface and the relative VBM energy for the Bi 2 Se 3 /GaAs interface from workfunction calculations of Δ=0.05 eV. Using these parameters, we fit the single parameter associated with the interaction α M =0.05 eV to produce the model band structure shown in Fig. 4b to compare with the ab initio band structure in Fig. 4a . Note that incorporation of the effect of interface roughness through a broadening of the interaction parameter in k -space, as outlined in ref. 17 , indicates that the results of the interaction are quite insensitive to the interface roughness, with gaussian broadening of 1.0 eV of the interaction parameter yielding differences in the band structure and spin textures of <0.1%. By analysing the spin textures of the first-principles calculations, we find that qualitative agreement can be reached when interaction is of the form V int ∝ σ z , and hence we set α 0 = α 1 = α 2 =0 and α 3 = i 0.05 eV. The spin texture of the model Hamiltonian is shown in Fig. 4d . The agreement of the features of bands b 2 and b 4 compare quite well between the calculation and model, being primarily right- and left-handed helical states, respectively, with the spin–momentum locking of both greatly diminished in the immediate vicinity of Γ. Bands b 1 and b 3 , however, appear less well described. While the nearly quenched spin–momentum locking of b 3 from ab initio calculation suggests that this band is less localized at the interface (and consequentially has less coupling), the origin of the deviation of b 1 from the model is clear. As we move away from Γ, the resulting decrease in the magnitude of spin is concurrent with the interaction of b 1 with lower-lying bands that are not considered in the model. The spin locking once again becomes more pronounced as the energy separation with lower-lying bands increases. This suggests that including more bands in the model will lead to a more quantitatively accurate description. Nonetheless, we note that the essential feature of the model is also found in the DFT calculation. That being that the top half of the Dirac cone, associated with left-handed helicity, and the bottom half of the Dirac cone, associated with right-handed helicity, are separated by an energy gap at Γ. To study the importance of the chemical treatments of the interface, we also investigated the electronic band structure and spin textures for the 1.00-ML Se-treated Bi 2 Se 3 /GaAs case. Since the 1.00-ML Se-treated GaAs surface is already metallic, the resulting interfacial dipole alters the alignment between Bi 2 Se 3 and GaAs. Note that, while in the case of 0.75 ML a VBM-derived state enters the bandgap and interacts with the Dirac cone, in the case of 1.00 ML, a metallic state comes down from the CBM to enter the gap, leading to a Δ of −0.10 eV (as opposed to 0.05 eV for the 0.75-ML case), as shown in the model calculation Fig. 5b . This modified Δ leads to a situation where bands b 3 and b 4 lie within the gap, but b 1 and b 2 are buried in the GaAs valence band, as can be seen in Fig. 5c , where the interfacial states have been highlighted in red. While this makes extracting the spin texture of b 1 and b 2 from first-principles calculations problematic, those of b 3 and b 4 are shown in Fig. 5d . These spin textures are well represented by the Hamiltonian model where the interaction has the same interaction strength found previously (0.05 eV), but the nature of the interaction is altered and it is paramterized by α 0 instead of the α 3 , which was found for the 0.75-ML case. Note that the other parameterizations predict a reversal of the helicity of the interfacial states at a critical | k |, see Fig. 2 , which is not observed in the case of 1-ML coverage. As such, interaction with the metallic CBM-derived state is fundamentally different from that of the insulating VBM-derived state, resulting in qualitatively different spin textures at the interface. 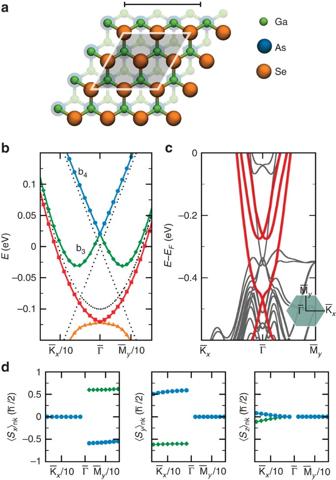Figure 5: First-principles calculations of electronic properties of 1.00-ML Se-treated Bi2Se3/GaAs. (a) Top view of a ball-and-stick model of a 1.00-ML Se-treated GaAs surface. Scale bar, 5 Å. (b) Effective model band structure for the interaction of the CBM-derived metallic state and the interfacial Dirac cone. (c) First-principles electronic band structure for the 1.00-ML Se-treated Bi2Se3/GaAs interface. The bands that are associated with the interface are highlighted in red. (d) First-principles spin texture of b3(green) and b4(blue) interface states. Figure 5: First-principles calculations of electronic properties of 1.00-ML Se-treated Bi 2 Se 3 /GaAs. ( a ) Top view of a ball-and-stick model of a 1.00-ML Se-treated GaAs surface. Scale bar, 5 Å. ( b ) Effective model band structure for the interaction of the CBM-derived metallic state and the interfacial Dirac cone. ( c ) First-principles electronic band structure for the 1.00-ML Se-treated Bi 2 Se 3 /GaAs interface. The bands that are associated with the interface are highlighted in red. ( d ) First-principles spin texture of b 3 (green) and b 4 (blue) interface states. Full size image The model presented in equation (1) and the finding of its applicability to realistic interfaces suggest that not only is the particle–hole symmetry of the Dirac cone fundamentally broken at the interface, but that a number of new emerging phenomena with potential applications exist. First, while optical excitations from linearly polarized light are spin forbidden for an ordinary Dirac cone, the spin interaction present at the interfacial Dirac cone relaxes this selection rule, leading to a number of allowed transitions, which generally become | k | dependent. This opens up the possibility of directly probing the topological interface states through optical means, such as absorption or photoluminescence. Furthermore, the well-delineated regions of different spin textures shown in Fig. 2 indicate the presence of a spin bottleneck, similar to the phonon bottleneck that limits the relaxation rates of hot carriers in graphene [21] , potentially leading to photosensitive conductivity and the prospect of the formation of an excitonic condensate at the interface. As electron relaxation into regions with a different spin texture would require a magnetic interaction, electron relaxation is now confined to individual shells of different spin textures with a prolonged excitation lifetime. Such a phenomenon should be observable for the Bi 2 Se 3 /GaAs interface with 0.75-ML Se coverage, which we predict to be the most stable Se-treated GaAs (111) surface under moderate Se availability, as shown in Fig. 3b . In this case, optical excitations to b 4 (shown in Fig. 4a ) for either from b 3 or lower-lying bands, will be long lived as electron relaxation down the b4 band requires spin modification. The resulting excess of carriers should be detectable as a persistent photoconductivity. In addition, this effect would be sensitive to magnetic perturbations, which could greatly reduce the lifetime of the excited carriers, and as such magnetic tuning of the lifetime of the persistent photoconductivity with an external magnetic field could firmly establish the existence of a spin bottleneck at the interface. In summary, we present a general and simple model to describe the interaction of the interfacial Dirac cone with non-topological states at the interface. This interaction is found to lead to a number of emerging phenomena, which highlight the differences between the Dirac cone at the surface of a TI and that found at the interface, including the vertical twinning of the Dirac cone, non-topological states acquiring spin texture and the reversal of the helicity of the Dirac cone. The main features of the model are demonstrated in our parameter-free density functional theory calculations of the Bi 2 Se 3 (0001)/GaAs(111) interface. The chemical details of Se treatment at the interface was found to profoundly alter the nature of the interaction between the TI and metallic CBM (insulating VBM)-derived semiconductor state, with the representative interaction proportional to ( σ 3 ) for the case of 1-ML(0.75 ML) coverage. The interaction proportional to σ 3 present for the 0.75-ML case results in clockwise–anticlockwise reversal of the helicity of the interfacial states at a critical | k |, pointing to altered optical selection rules and prolonged excitation lifetimes. While we have focused on the interaction of the emerging Dirac cone with bulk-derived states at the TI/NI interface, the model is more general and could be trivially extended to investigate the interactions of the surface Dirac cone with other non-topological states. These findings both suggest a new possible phenomenon at the interface and may help to guide developments in TI/NI-based spintronics devices, especially due to the helical topological states’ role in spin current generation [11] , [14] and spin relaxation [15] . Density functional theory The atomistic first-principles calculations were performed within the DFT framework [22] , [23] as implemented in the Vienna Ab Initio Simulation Package [24] , [25] . Energy cutoff of 300 eV and k -point grid of 3 × 3 × 1 in Monkhorst—Pack algorithm [26] were taken as default in our calculations. Interactions between ion cores and valence electrons are described by the projector-augmented wave method [25] , [27] . The exchange-correlation functional was in local density approximation [28] parameterized by Perdew—Zunger [29] due to agreement with experimental bond lengths among Bi 2 Se 3 quintuple layers [30] . Electronic band structures and spin textures required non-collinear spin polarizations for spin–orbit interactions. The chemical stability of Se on the isolated As-terminated GaAs(111) surface was determined by slab calculations in a 2 × 2-unit cell with 18 atomic layers. The Ga-terminated surface was passivated with H with a fractional charge ( q =1.25 e ). To minimize the effect of strain, a lattice constant of 4.07 Å was used in the interface calculation. The stacking with the Se atomic layer of Bi 2 Se 3 directly above the H3 substrate was chosen as it was found to be 20 and 490 meV per supercell lower in energy than the T4 and T1 configurations, respectively. How to cite this article: Seixas, L. et al. Vertical twinning of the Dirac cone at the interface between topological insulators and semiconductors. Nat. Commun. 6:7630 doi: 10.1038/ncomms8630 (2015).